3-sulfonyloxyaryl(mesityl)iodonium triflates as 1,2-benzdiyne precursors with activation viaortho-deprotonative elimination strategy Benzyne has long captivated the attention of chemists and has gained numerous synthetic achievements. Among typical benzyne generation methods, removal of two vicinal substituents from 1,2-difunctionalized benzenes, i.e., Kobayashi’s protocol, are prevailing, while ortho -deprotonative elimination from mono-substituted benzene lags far behind. Despite the advantages of atom economy and ready achievability of precursors, a bottle neck for ortho -deprotonative elimination strategy resides in the weak acidity of the ortho -hydrogen, which normally demands strong bases as the activating reagents. Here, an efficient aryne generation protocol is developed, where ortho -deprotonative elimination on 3-sulfonyloxyaryl(mesityl)iodonium triflates occurs under mild conditions and the generated 3-sulfonyloxyarynes can serve as efficient 1,2-benzdiyne synthons. This array of 1,2-benzdiyne precursors can be conveniently prepared with high functional group tolerance, and densely substituted scaffolds can be accessed as well. Carbonate and fluoride salts are found to serve as efficient activating reagents, which are the weakest bases used in ortho -deprotonative elimination strategies. Particularly, this scaffold has predictable chemoselective generation of the designated aryne intermediates. The success of this ortho -deprotonative elimination protocol sets up a unique platform with a broad spectrum of synthetic applications. A distinct property of benzyne chemistry is the ready assembly of two vicinal chemical bonds in step-economical manner [1] , [2] , [3] . Along with the extensive application of mild generation methods in the past two decades, i.e., Kobayashi’s protocol [4] and via hexadehydro-Diels-Alder (HDDA) reactions [5] , numerous benzyne transformations have been unraveled [5] , [6] , [7] , [8] , [9] , [10] , [11] , [12] , [13] , [14] , [15] , [16] , [17] , [18] , [19] , [20] . Due to the fleeting character of a benzyne species, however, it has to be generated in situ from a precursor and, preferentially, via a slow releasing manner. Consequently, both the constitution of a benzyne precursor and its generation conditions are essential for the success of a benzyne-engaged transformation. In this context, efforts to explore new generation methods have been accompanied with the development of benzyne chemistry. To date, there are two major strategies to generate benzyne, either removal of two vicinal substituents from 1,2-difunctionalized benzene or ortho -deprotonative elimination from mono-substituted benzene. Between these two strategies, ortho -disubstituted benzyne precursors have been recognized as the most popular ones, primarily due to their ease to be activated and the accommodation of the generated benzyne to various types of reactions. For instance, o -silylaryl triflates (Kobayashi’s aryne precursors) have been the most utilized precursors in the past two decades and are accounted for the recent renaissance of benzyne chemistry [20] . Despite the facts that ortho -deprotonative elimination strategy was first used in the early era of benzyne chemistry and possesses its merit by removing only one leaving group (LG) along with deprotonation, it is now lagging far behind of the current prevailing strategy employing 1,2-disubstituted benzyne precursors. Presumably, a marked obstacle for ortho -deprotonative elimination strategy is the weak acidity of the ortho -proton of typical leaving groups, which remains to be a challenge in benzyne chemistry. Since 1940s, strong bases, such as phenyllithium and NaNH 2 , have been employed to deprotonate halobenzenes (Fig. 1a ) [20] . In 1991, phenyl triflate was used as the precursor, where lithium diisopropylamide (LDA) served as both the activating reagent and nucleophile [21] . To avoid unwanted nucleophilic addition by the base, lithium 2,2,6,6-tetramethylpiperidide (LiTMP) [22] , [23] , [24] , [25] , [26] , lithium diadamantylamide (LDAM) [27] , and lithium di-alkyl(2,2,6,6-tetramethylpiperidino)zincate (R 2 Zn(TMP)Li) were successfully developed [28] , [29] . Alternatively, diaryliodonium salts were reported first by Akiyama in 1974 [30] and recently revisited by Stuart [31] , [32] , [33] , [34] to serve as aryne precursors. The advantage for this generation method is based on the fact that the hypernucleofugality of aryliodonio group is million-time better than that of OTf group [35] . However, those strong bases and organometallic reagents used in the aryne generation step fall short of functional group compatibility, which also limit the discovery of benzyne transformations. Very recently, cyclic diaryl λ 3 -bromanes/λ 3 -chloranes were found to serve as aryne precursors, where Cs 2 CO 3 could efficiently deprotonate the ortho -hydrogen to generate the corresponding arynes due to the better leaving tendency of λ 3 -bromane/ λ 3 -chloranes than that of hypervalent iodide [36] , [37] , [38] . The mechanistic study also revealed that deprotonation and C-X bond cleavage should be a concerted process via seven-membered cyclic transition state involving carbonate anion [38] . Although promising, this method is limited to cyclic λ 3 -bromanes and only bromo-biaryl compounds were obtained, where the application of acyclic λ 3 -bromanes was restricted due to the high reactivity of BrF 3 that is normally used to prepare acyclic λ 3 -bromanes through ligand exchange [39] . Fig. 1: Background and our work. a Timeline of ortho -deprotonative elimination protocols. b Problems associated with the application of previous domino 1,2-benzdiyne precursors. TPBT: 2-(trimethylsilyl)−1,3-phenylene bis(trifluoromethanesulfonate). TTPM: 3-(((trifluoromethyl)sulfonyl)oxy)−2-(trimethylsilyl)phenyl 4-methylbenzenesulfonate. TTPF: 3-(((trifluoromethyl)sulfonyl)oxy)−2-(trimethylsilyl)phenyl 2,6-difluorobenzenesulfonate. c Our work. Full size image In the past a few years, we spent our effort on 1,2-benzdiyne transformations, where polysubstituted arenes containing biologically active frameworks could be conveniently prepared either via tandem processes or in stepwise manner [18] , [40] , [41] , [42] , [43] , [44] , [45] , [46] , [47] . A series of domino aryne precursors based on 2-silylaryl 1,3-bis(sulfonate) framework were developed along with our study (Fig. 1b ). Although possessing promising potential, the employment of Kobayashi’s benzyne generation method in our 1,2-benzdiyne system lacks functional group economy. Moreover, two notable restrictions exist to prevent this structural motif from reaching unsymmetrically substituted precursors and/or reaction products. On one hand, it cannot manipulate site-selective generation of 4- or 6-substituted 3-triflyloxybenzyne (intermediate i vs ii , Fig. 1b ) from TPBT-based framework [43] . On the other hand, it is hard to access either 4- or 6-functionalized TTPM/TTPF-based scaffold from unsymmetrically substituted resorcinols due to limited sources of feedstocks as well as the lack of practical method to differentiate two OH groups on them. As a result, only several substituted TPBTs and TTPMs were reported so far [18] . In this context, an emerging need is to judiciously redesign structures of 1,2-benzdiyne equivalents so that a broad range of precursors could be conveniently accessed and a variety of densely substituted arenes bearing potential biological properties can be conceived after 1,2-benzdiyne transformations. We envisioned that those building blocks that could utilize ortho -deprotonative elimination strategy to trigger 1,2-benzdiyne transformations under mild conditions would be more appropriate and practical candidates. To this end, we proposed the following criteria for 1,2-benzdiyne equivalents: (1) mild activation conditions, i.e., with weak base and activation temperature ranging from 0 o C to 100 o C, via ortho -deprotonative elimination strategy that possess the advantage of functional group economy; (2) ready preparation for substituted analogues; (3) site-selective generation of the designated aryne upon activation. In our previous studies on 1,2-benzdiyne transformations, carbonate salts were found to efficiently kick out the trimethylsilyl (TMS) group on those precursors in Fig. 1b , the weakened C(aryl)-Si bond of which should be the result of the σ -electron-withdrawing ( σ -EW) effect of two ortho -sulfonate groups. Moreover, both Tilley [48] and Stuart [31] , [32] , [33] , [34] observed the site-selective generation of arynes via ortho -deprotonative elimination pathways, which are consistent with the calculation on proximity-induced acidity of C2-hydrogen [49] . In this context, we postulated that as long as the sum of σ -EW effect is large enough, the acidity of this C2-H might eventually reach the level to be deprotonated by weak bases. Since many σ -EW groups are LGs as well, 1,2-benzdiyne equivalents would be conceived. Herein, we wish to report our discovery on a mild ortho -deprotonative elimination protocol to initiate 1,2-benzdiyne transformations from 3-sulfonyloxyaryl(mesityl)iodonium triflates, in which carbonate and even fluoride salts could serve as efficient activating reagents (Fig. 1c ). This scaffold has a substantially expanded precursor scope with preferential generation of substituted 3-sulfonyloxyarynes due to the superb leaving tendency of the mesityliodonio group. Initial tests To probe our hypothesis, we first examined 1,3-phenylene bis(trifluoromethanesulfonate) ( 1a ) in order to see whether 3-triflyloxybenzyne i could be generated in the presence of carbonate (Fig. 2a ). Unfortunately, no [4 + 2]-cycloadduct 2a with furan was detected in this reaction and 90% of 1a was recovered, suggesting that its C2-hydrogen is not acidic enough. Inspired by the observation that aryliodonio group is a much better LG than OTf [35] , [50] , we decided to prepare and examine compound 1b by introducing a mesityliodonium salt at the meta -position of the OTf group (Fig. 2b ). Expectedly, the enhanced acidity of the C2-H in response to the presence of two proximal strong σ -EWGs, namely an OTf and an aryliodonio group, could eventually allow its deprotonation by carbonates. As shown in eq 2, the preparation of compound 1b followed a one-pot oxidation protocol from 3-iodophenyl triflate ( 3a ) [51] . Upon activation with Cs 2 CO 3 /18-c-6 in acetonitrile, gratifyingly, 2a was obtained in 64% yield. Fig. 2: Initial studies. a The reaction between 1a and furan in the presence of carbonate salts furnished no desired cycloadduct 2a . b The preparation of 1b and its reaction with furan in the presence of Cs 2 CO 3 gave rise to cycloadduct 2a in 64% yield. Full size image Reaction optimization Encouraged by this preliminary result, we decided to optimize this transformation. 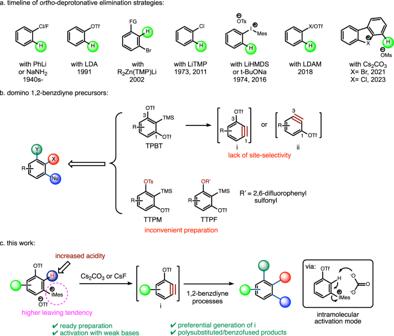Fig. 1: Background and our work. aTimeline ofortho-deprotonative elimination protocols.bProblems associated with the application of previous domino 1,2-benzdiyne precursors. TPBT: 2-(trimethylsilyl)−1,3-phenylene bis(trifluoromethanesulfonate). TTPM: 3-(((trifluoromethyl)sulfonyl)oxy)−2-(trimethylsilyl)phenyl 4-methylbenzenesulfonate. TTPF: 3-(((trifluoromethyl)sulfonyl)oxy)−2-(trimethylsilyl)phenyl 2,6-difluorobenzenesulfonate.cOur work. By varying solvents, DCM was found to be a comparable one with acetonitrile (entry 4, Table 1 ). Unexpectedly, the absence of 18-c-6 in the reaction media could substantially increase the yield of 2a in both DCM and acetonitrile (entries 5 and 6), despite the fact that Cs 2 CO 3 has low solubility in both solvents. This observation could be explained by the fact that the cationic diaryliodonium ion itself might help dissolve carbonate through ligand exchange [52] . Consequently, intramolecular deprotonation on C2-podition would occur to allow a smooth generation of 3-triflyloxybenzyne i under mild conditions (Fig. 1c ) [38] . By contrast, Ochiai et al. reported that 18-c-6 was found to coordinate with aryliodonio groups and, hence, decreases its leaving ability [53] . Next, it was found that K 2 CO 3 featured 2a in slightly diminished yield (entry 7). Interestingly, while the employment of CsF furnished 2a in only 52% yield at room temperature, this yield could raise to 77% when the reaction was carried out at 70 o C in a sealed tube (entry 8). Notably, these activating reagents in our study, efficiently with Cs 2 CO 3 and even effectively with CsF, are the weakest bases so far through ortho -deprotonative elimination strategy [20] . The prominent advantages by employing these weak inorganic bases as the activating reagents are both compatibility to various tandem reaction processes and excellent functional group tolerance as have been proven in our previous studies. In comparison, the absence of base gave no generation of 3-triflyloxybenzyne i at all (entry 9). Table 1 Optimization of reaction conditions Full size table In addition to 1b , we also prepared compounds 1c and 1d containing 3-sulfonyloxy groups other than OTf group (entries 10 and 11, Table 1 ). When compound 1c bearing a 3-OTs group was employed, its reaction with furan afforded 2b in 63% yield. Notably, compound 1c can be seen as the structural analogue of 1,2-benzdiyne precursor TTPM (Fig. 1b ) [45] . Similarly, compound 1d containing a 2,6-difluorophenylsulfonate group at the C3-position is an analogue of TTPF (Fig. 1b ) [47] , and its reaction with furan gave rise to the corresponding [4 + 2]-cycloadduct 2c in 66% yield. Notably, compounds 1b - 1d are bench-stable white solid and do not decompose at room temperature for several months, making them appropriate 1,2-benzdiyne reagents. Substrate scope The ready accessibility of functionalized 3-iodophenyl triflates 3 either from commercial feedstocks or via typical manipulations on them allows the convenient synthesis of this array of 1,2-benzdiyne precursors 1 . Along with our study, several practical preparation protocols toward 3-iodophenyl triflates 3 were developed: (a) diazotization-iodination and triflation of substituted 3-aminophenols; (b) meta -nitration of para -alkylated phenyl triflate/reduction/diazotization-iodination; (3) para -nitration of aryl triflate/reduction/ ortho -iodination of aniline/diazotization-reduction (please see the Supplementary Information (SI) for details). After accessing these substituted 3-iodophenyl triflates 3 , a series of 1,2-benzdiyne precursors 1e - 1t were readily synthesized upon oxidation with either m -CPBA [51] or Oxone [54] using one-pot oxidation protocols (Fig. 3a ). Those substituents can be alkyl, halo, ester, trifluoromethyl, and triflyloxy groups. In addition, two pairs of benzofused analogues 1u - 1x were obtained. Depending on the location of the mesityliodonio group, different substituted 3-triflyloxybenzyne intermediates could be envisioned in each pair. Furthermore, penta-substituted aryne precursors 1 y and 1z were prepared as well. It is worth mentioning that upon activation the corresponding arynes from compounds 1u - 1z are otherwise difficult to be reached from 2-silylaryl 1,3-bis(sulfonate) skeleton (Fig. 1b ). Besides, 2,3-pyridiyne equivalent 1aa and 3,4-pyridiyne equivalent 1bb were successfully achieved. Fig. 3: Scope for domino aryne precursors. a Scope with classical preparation method. b Preparation of electron-rich substrates using Kita’s approach. c Preparation of TTPM/TTPF-based scaffold. Reaction conditions: [a] A solution of 3 (1.0 mmol), m -CPBA or Oxone (1.5 mmol), triflic acid (2.0 mmol) in solvent (5.0 mL) was stirred from 0 o C to rt for 3 hours; mesitylene (1.1 mmol) was then added. [b] Isolated yield. [c] A solution of 4 (0.22 mmol) and PhI(OH)OTs 5 (0.2 mmol) in 2,2,2-trifluoroethanol (2 mL) was stirred at rt. [d] The reaction was carried out in DCM (2 mL) with NaOTf (1.0 mmol). [e] A solution of 3′ (1.0 mmol), m -CPBA or Oxone (1.5 mmol), triflic acid (2.0 mmol) in solvent (5.0 mL) was stirred from 0 o C to rt for 3 hours; mesitylene (1.1 mmol) was then added. Full size image We noticed that those substituents on 1,2-benzdiyne precursors in Fig. 3a are either alkyl groups or EWGs. Because electron-rich arenes could compete with mesitylene in the formation of diaryliodonium salt step, strong electron-donating groups (EDGs) were found to be incompatible with the reaction conditions through the above oxidation protocols. In order to incorporate EDGs onto the parent benzene ring, we decided to employ Kita’s approach, where direct dehydrative condensation of electron-rich arenes with PhI(OH)OTs ( 5 ) (Koser’s reagent) could occur in fluoroalcohol media [55] . As shown in Fig. 3b , the reaction of 2-methoxyphenyl triflate with Koser’s reagent in 2,2,2-trifluoroethanol featured compound 1cc regioselectively in 82% yield. Activation of 1cc with Cs 2 CO 3 in DCM in the presence of furan could furnish the desired [4 + 2]-cycloadduct, confirming that the newly introduced phenyliodonio group on 2-methoxyphenyl triflate is on the meta -position of the OTf group. Similarly, compounds 1dd - 1gg were readily prepared using this method and the 2-methoxy group serves as an efficient directing group to regulate the incorporation of phenyliodonio group onto the C5-position exclusively. Moreover, 2-silyl group on p -methoxyphenyl triflate was found to tolerate the reaction conditions, furnishing compound 1hh in 60% yield. Notably, compound 1hh could also be seen as 1,3-benzdiyne equivalent, where chemoselective generation of the designated 3-triflyloxyaryne intermediate should occur. At last, compound 1ii was also obtained, albeit in only 30% yield. By using this protocol, a series of aryne precursors containing strong electron-donating groups were obtained. Our previous studies revealed that the leaving ability of the second leaving group on domino aryne precursors has profound influence to the efficiency of these reagents in various cascade processes, such as nucleophilic-ene reactions as well as nucleophilic and Diels-Alder cycloaddition reactions [18] . Consequently, those domino aryne precursors containing either an OTs group (TTPM) or a 2,6-difluorophenylsulfonyloxy (OFPs) group (TTPF) were found to be more appropriate ones than TPBT with two OTf groups. Therefore, it is desirable to find an approach to prepare those alternative yet indispensable aryne precursors containing either an OTs or an OFPs group. Since triflation of phenols belongs to one of the early steps in the preparation of many aryne precursors in Fig. 3a , a direct conversion of the OTf group to either OTs or OFPs group on 3-iodoaryl triflates 3 could provide a divergent solution and would be highly desirable. Pleasingly, by employing Nishiyama’s protocol [56] , deprotection of the OTf group on 3-iodoaryl triflates 3 with tetrabutylammonium hydroxide (Bu 4 NOH) in 1,4-dioxane was realized in quantitative yield. Upon one-pot protection with sulfonyl chloride, 3-iodoaryl sulfonates 3 ′ were furnished (Fig. 3c ). As such, we chose those iodobenzenes 3 that were used to prepare 1s - 1z , because these scaffolds are tetra- and pentasubstituted benzenes and could result in the formation of densely substituted arenes through domino aryne transformations. After oxidation of 3 ′, compounds 1s-Ts - 1z-Ts as analogues of 1c and 1s-FPs - 1z-FPs as analogues of 1d could be prepared (Fig. 3c ). The expeditious preparation of those 1,2-benzdiyne precursors in Fig. 3 sets up a general and potentially useful platform for 1,2-benzdiyne study. Synthetic applications After successfully prepared those 1,2-benzdiyne precursors, we set out to examine their reactivity in tandem 1,2-benzdiyne transformations in order to see whether this scaffold is compatible with different aryne reaction conditions. As shown in Fig. 4 , the reactions of 1b - 1d with various substrates were tested. First, the reaction of 1b with pivaloyl (Piv)-protected benzothioamide 6 afforded benzothiazole 7a in 77% yield. Moreover, 1,3-diaminobenzene 9 could be produced in 78% yield by treating N -triflated aniline 8 with 1b in acetonitrile at room temperature. Similarly, 1,2-diamination reaction with sulfonamide 10 took place to furnish 11 in 56% yield. Besides, electron-deficient p -cyanophenol 12 was found to serve as efficient nucleophile, featuring diaryl ether of resorcinol 13 in 65% yield. Notably, phenols have not yet been employed in our domino aryne transformations. Next, tandem nucleophilic-ene reactions of aryne precursor 1c with tosylamides 14 and 16 were examined. As have been disclosed that aryne precursor TTPM bearing an OTs leaving group was mandatory for the success of this transformation, because the departure rate of the OTs group matches well with that of the intramolecular ene reaction. Indeed, when aryne precursor 1c was employed using the standard conditions (chlorobenzene at 130 o C) in our previous study [45] , the corresponding products 15a and 17 were achieved, respectively, in good yields. At last, cascade nucleophilic and Diels-Alder reactions were examined [47] . Unexpectedly, the reaction of 1c with cinnamyl amide 18 could feature 19a in only 36% yield using chlorobenzene at 130 o C. Gratifyingly, by employing 1d bearing an OFPs group and using toluene-MeCN as binary solvent system, tetracyclic compound 19a was obtained in 72% yield. This observation indicates that the OFPs group on 1d is more appropriate than the OTs group on 1c in this tandem nucleophilic and Diels-Alder reaction process, which is different from our previous domino aryne system in the same transformation [47] . The examples in Fig. 4 clearly illustrated that our 1,2-benzdiyne scaffold has comparable efficiency with those using 2-silylaryl 1,3-bis(sulfonate) skeleton. Fig. 4: Study on domino aryne reactions with 1b-1d. All reactions are performed on a 0.2 mmol scale. Isolated yields are given. Full size image Beyond mild generation conditions, another distinct advantage for this array of 1,2-benzdiyne precursors is the predictability in both the site-selective generation of 1,2-aryne intermediate and the subsequent aryne reactions. Because of the better-leaving tendency of the aryliodonio group than that of the sulfonyloxy group, 3-sulfonyloxyaryne intermediate iii should be always generated preferentially upon deprotonation with base (Fig. 5 ). Since sulfonyloxy groups are σ -EWGs, they could direct the incoming nucleophile to attack their meta -positions to release 2,3-aryne iv (Fig. 5 ). Consequently, unsymmetrically substituted 3-sulfonyloxyarynes iii would then be converted to the corresponding products via domino aryne processes in regioselective manner. To demonstrate this property, aryne precursors 1s - 1z containing two or more additional substituents were chosen for our study. It was envisioned that heavily substituted arenes should be achieved via different domino aryne transformations. Fig. 5: Preparation of densely functionalized arenes. a Cascade reactions with 6 . b Cascade nucleophilic-one reactions with 14 . c Cascade nucleophilic, [4 + 2]-cycloaddition reactions with 18 . d Reactions with N -benzoylbenzamide. Reaction conditions: [a] Slow addition of a solution of 1 (0.4 mmol) in 1,4-dioxane (3 mL) to a suspension of benzothioamide 6 (0.2 mmol), Cs 2 CO 3 (1.6 mmol), and 18-c-6 (0.4 mmol) in 1,4-dioxane (3 mL) at 80 o C over 3 hours. 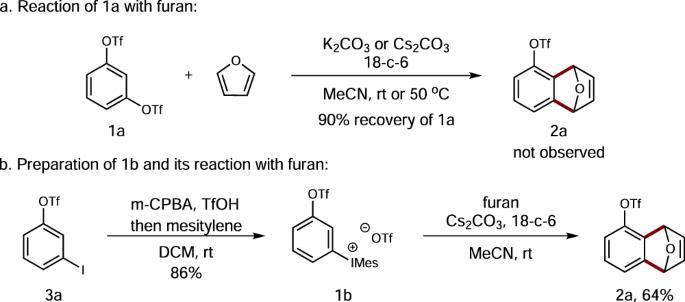Fig. 2: Initial studies. aThe reaction between1aand furan in the presence of carbonate salts furnished no desired cycloadduct2a.bThe preparation of1band its reaction with furan in the presence of Cs2CO3gave rise to cycloadduct2ain 64% yield. [b] Slow addition of a solution of 1-TS (0.4 mmol) in chlorobenzene (3 mL) to a suspension of tosylamide 14 (0.2 mmol), Cs 2 CO 3 (1.6 mmol), and 18-c-6 (0.4 mmol) in chlorobenzene (3 mL) at 130 o C over 3 hours. [c] Slow addition of a solution of 1-FPs (0.4 mmol) in MeCN (7 mL) to a suspension of cinnamyl amide 18 (0.2 mmol), Cs 2 CO 3 (1.2 mmol), and 18-c-6 (0.1 mmol) in toluene (7 mL) at 100 o C over 4 hours. [d] Slow addition of a solution of 1 (0.8 mmol) in acetonitrile (5 mL) to a suspension of N -benzoylbenzamide (0.4 mmol), Cs 2 CO 3 (1.6 mmol), water (0.08 mmol), and 18-c-6 (0.2 mmol) in acetonitrile (5 mL) at 80 o C over 8 hours. Full size image We first examined the reactions between benzothioamide 6 and aryne precursors 1s - 1z . Penta-substituted benzothiazoles 7b - 7g and hexa-substituted benzothiazoles 7h and 7i were obtained in moderate to good yields. Notably, topological isomers 7d and 7e were prepared in regiospecific manner from 1u and 1v , respectively (Fig. 5a ). Similar results were also observed with respect to 7f and 7g as well as 7h and 7i , those of which were exclusively derived from their corresponding 1,2-benzdiyne precursors. Distinctively, complementary regioselective control could be realized through the employment of this 1,2-benzdiyne scaffold. Next, tandem nucleophilic-ene reactions of 14 with aryne precursors 1s-Ts - 1z-Ts were studied, featuring the corresponding indoline products 15b - 15g and 15i in moderate to high yields (Fig. 5b ). However, it was found that compound 15h was achieved in only 10% yield from 1y-Ts . Gratifyingly, when aryne precursor 1y-FPs was employed, its reaction with 14 in toluene-MeCN binary solvent was able to deliver 15h in 56% yield. At last, cascade nucleophilic and Diels-Alder reactions with cinnamyl amide 18 were tested. As shown in Fig. 5c , its reactions with 1s-FPs - 1z-FPs could readily construct tetra- and pentacyclic ring systems 19b - 19i . These examples revealed that our 1,2-benzdiyne precursors should find a broad spectrum of synthetic applications, where both heavily substituted arenes and benzofused polycyclic ring systems with diverse substitution patterns could be accomplished. Particularly, those structures containing benzothiazole, indoline, and benzofused [6,5,6,6]-tetracyclic ring system possess potential biological activity, which are otherwise almost incapable to access through 2-silylaryl 1,3-bis(sulfonate) framework. Besides, a reactivity of domino aryne system was discovered with this set of precursor scaffold. As shown in Fig. 5d , the reaction of aryne precursor 1b with N -benzoylbenzamide gave rise to the formation of benzoxazole 20a in 68% yield. This reaction is apparently different from that with benzothioamide 6 [40] , in which the benzoyl group does not migrate to the 3-position of the parent aryne ring. When aryne precursor 1e was employed, a mixture of 20b and 20b’ was obtained in 49% yield with a 3:1 ratio, illustrating that both the nitrogen and the oxygen on N -benzoylbenzamide could serve as the first nucleophile to attack the generated 3-triflyloxybenzyne intermediate. By employing 1w and 1u as the aryne precursors, the corresponding benzoxazoles 20c and 20d were achieved, respectively, in moderate yields. In addition, we also carried out preliminary investigations on pyridiyne equivalents. As shown in Fig. 6 , 3,4-pyridiyne precursor 1bb was first examined. Its reaction with benzothioamide 6 could furnish benzothiazole 21a in 61% yield. Moreover, both 1,3-diamination and 1,2-diamination were tested, and 21b and 21c were obtained in moderate yields (Fig. 6 ). Unfortunately, efforts to apply both tandem nucleophilic-ene reaction as well as nucleophilic and [4 + 2]-cycloaddition processes failed to produce the desired products at all, suggesting that 3,4-pyridiyne precursor 1bb has different reaction behavior comparing with its 1,2-benzdiyne counterpart 1b . When 2,3-pyridiyne precursor 1aa was treated with various arynophiles, only complex mixtures were observed with no formation of the desired 2,3-pyridiyne reaction products. Fig. 6: Study on pyridiyne precursor 1bb. All reactions are performed on a 0.2 mmol scale. Isolated yields are given. Full size image Next, we wanted to see whether this 1,2-benzdiyne scaffold could be applied in the [2 + 2]-cycloaddition, Grob-fragmentation process previously developed by our group [44] . As shown in Fig. 7 , we chose aryne precursors 1 u and 1 v in our study. First, formal [2 + 2]-cycloaddition of 1 u with ketene silyl acetal (KSA) 22a (R’ = Me) could afford cycloadduct 23a in 50% yield in regioselective manner. Similarly, compound 23b was obtained in 85% yield from 1 v and 22b (R’ = H) as well. 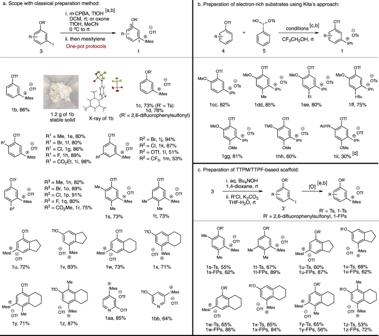Fig. 3: Scope for domino aryne precursors. aScope with classical preparation method.bPreparation of electron-rich substrates using Kita’s approach.cPreparation of TTPM/TTPF-based scaffold. Reaction conditions: [a] A solution of3(1.0 mmol),m-CPBA or Oxone (1.5 mmol), triflic acid (2.0 mmol) in solvent (5.0 mL) was stirred from 0oC to rt for 3 hours; mesitylene (1.1 mmol) was then added. [b] Isolated yield. [c] A solution of4(0.22 mmol) and PhI(OH)OTs5(0.2 mmol) in 2,2,2-trifluoroethanol (2 mL) was stirred at rt. [d] The reaction was carried out in DCM (2 mL) with NaOTf (1.0 mmol). [e] A solution of3′(1.0 mmol),m-CPBA or Oxone (1.5 mmol), triflic acid (2.0 mmol) in solvent (5.0 mL) was stirred from 0oC to rt for 3 hours; mesitylene (1.1 mmol) was then added. It is worth mentioning that in our previous study the reaction between TPBT and KSAs 22 gave no [2 + 2]-cycloaddition products at all [44] , suggesting that 3-sulfonyloxyaryl(mesityl)iodonium triflates are more amenable to [2 + 2]-cycloaddition reactions than TPBT-based framework. With both tricyclic compounds 23a and 23b in hand, we then selected several arynophiles to capture the 2,3-aryne intermediates generated upon activation with CsF in acetonitrile. The reaction of 23a with imidazole gave the nucleophilic addition product 24a as a single isomer in 57% yield. Meanwhile, its reaction with benzyl azide furnished a [3 + 2]-cycloadduct 24b in 63% yield in excellent regioselectivity. On the other hand, the reactions of cycloadduct 23b with either nitrone or furan produced the corresponding cycloadducts 24c and 24d in excellent yields, both of which are pentasubstituted arenes. In view of the potential of this two-step process in accommodating a variety of arynophiles as well as reaction modes, diverse patterns of densely substituted arenes could be foreseen by combining this process with these 1,2-benzdiyne precursors. Fig. 7: Manipulation through [2 + 2]-cycloaddition, Grob-fragmentation processes. All reactions are performed on a 0.4 mmol scale. Isolated yields are given. Full size image In order to demonstrate the potential of our domino aryne system, particular those bearing 3-sulfonyloxyaryl(mesityl)iodonium triflate structural motif, we carried out a synthesis toward natural products (±)-esermetole and (±)-physostigmine [57] , [58] , [59] . As shown in Fig. 8 , the Wittig reaction between 1-hydroxypropan−2-one and ethyl 2-(triphenyl- λ 5 -phosphaneylidene)acetate, followed by Mitsunobu reaction with tert -butyl tosylcarbamate ( p -TsNHBoc), could furnish compound 25 in 55% yield over two steps. Next, sequential reduction, O-methylation, and deprotection on compound 25 delivered compound 26 in 78% yield in a one-pot, three-step fashion. Meanwhile, aryne precursor 1cc-FPs was readily prepared from 2-methoxyphenol using the Kita’s approach (Fig. 3b ). The key step for domino aryne nucleophilic-ene reaction between 1cc-FPs and compound 26 in toluene-acetonitrile binary solvent system could furnish compound 27 in 60% yield. In this transformation, we noticed that the second leaving group on the domino aryne precursor framework is essential to allow acceptable level of reaction efficiency. 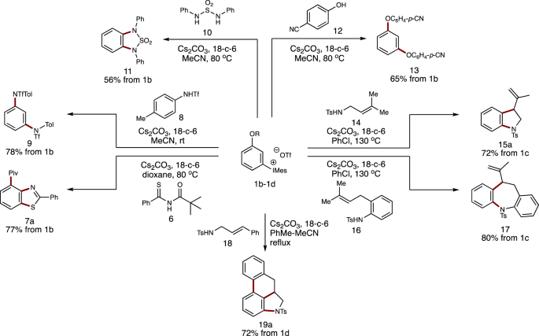Fig. 4: Study on domino aryne reactions with 1b-1d. All reactions are performed on a 0.2 mmol scale. Isolated yields are given. In comparison, aryne precursors containing either an OTf group ( 1cc ) or an OTs group ( 1cc-Ts ) on the 3-position only resulted in the formation of compound 27 in low yield. By contrast, it is difficult to prepare the corresponding domino aryne precursor containing 4-methoxy group based on the TTPM/TTPF framework and there will be no site selective activation upon aryne generation from TPBT-based scaffold (Fig. 1b ). Therefore, the construction of compound 27 demonstrates a great potential of this type of 1,2-benzdiyne scaffold in synthesizing a broad range of useful molecules containing functionalized arenes. Next, deprotection of the tosyl group on compound 27 with sodium-naphthalene solution in THF furnished compound 28 in 65% yield, which was followed by oxidation of 28 with manganese dioxide to feature compound 29 in 40% yield. Subsequent N-methylation and conversion of the enol methyl ether to aldehyde could be realized in one-pot fashion to afford compound 30 in 90% overall yield. It has been reported that compound 30 would then be transformed to (±)-esermetole and (±)-physostigmine according to literature precedents [57] , [58] , [59] . Fig. 8: Study toward the synthesis of (±)-esermethole and (±)-physostigmine. A preparation of compound 30 was realized by employing domino aryne nucleophilic-ene reaction between aryne precursor 1cc-FPs and compound 26 as the key step. After obtaining compound 27 , subsequent deprotection, oxidation, N-methylation, and conversion of the enol methyl ether to aldehyde gave rise to the desired compound 30 . Isolated yields are given. Full size image In summary, a class of 1,2-benzdiyne precursors were successfully developed by employing ortho -deprotonative elimination strategy as the generation method under mild conditions. A broad range of precursors with various substituents on the parent arene ring, including benzofused scaffolds as well as heavily functionalized analogues, could be conveniently prepared. Distinctively, weak bases, such as carbonate and even fluoride salts, were found to serve as efficient activating reagents, which are the weakest bases used in ortho -deprotonative elimination strategies so far. As an exhibition, a broad spectrum of intensely functionalized arenes as well as polycyclic ring systems were achieved, those of which contain potential biological properties. This protocol represents a breakthrough in 1,2-benzdiyne chemistry with high functional group compatibility as well as excellent chemoselective control upon activation. In a broader context, our study refreshes the traditional understanding that ortho -deprotonative elimination strategies normally require strong bases to realize deprotonation task and, hence, have been limited in only a few types of aryne transformations. It can be envisioned that this array of 1,2-benzdiyne precursors not only provide a convenient maneuver to access various substituted analogues, but also could be used in the exploration of unexplored aryne/domino aryne transformations. General procedure for the transformation of aryl triflate to aryl tosylate or aryl 2,6-difluorophenylsulfonate To a solution of 3-iodoaryl triflate (1.0 mmol, 1.0 equiv) in 1,4-dioxane (20 mL) at room temperature was added 40% aq. Bu 4 NOH (1.33 mL, 2.0 mmol, 2.0 equiv). 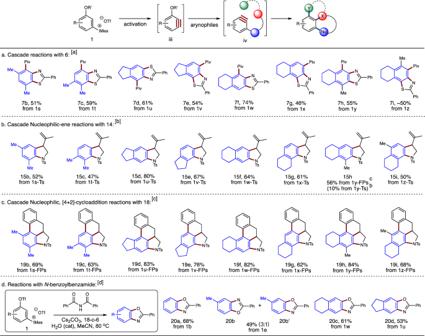Fig. 5: Preparation of densely functionalized arenes. aCascade reactions with6.bCascade nucleophilic-one reactions with14.cCascade nucleophilic, [4 + 2]-cycloaddition reactions with18.dReactions withN-benzoylbenzamide. Reaction conditions: [a] Slow addition of a solution of1(0.4 mmol) in 1,4-dioxane (3 mL) to a suspension of benzothioamide6(0.2 mmol), Cs2CO3(1.6 mmol), and 18-c-6 (0.4 mmol) in 1,4-dioxane (3 mL) at 80oC over 3 hours. [b] Slow addition of a solution of1-TS(0.4 mmol) in chlorobenzene (3 mL) to a suspension of tosylamide14(0.2 mmol), Cs2CO3(1.6 mmol), and 18-c-6 (0.4 mmol) in chlorobenzene (3 mL) at 130oC over 3 hours. [c] Slow addition of a solution of1-FPs(0.4 mmol) in MeCN (7 mL) to a suspension of cinnamyl amide18(0.2 mmol), Cs2CO3(1.2 mmol), and 18-c-6 (0.1 mmol) in toluene (7 mL) at 100oC over 4 hours. [d] Slow addition of a solution of1(0.8 mmol) in acetonitrile (5 mL) to a suspension ofN-benzoylbenzamide (0.4 mmol), Cs2CO3(1.6 mmol), water (0.08 mmol), and 18-c-6 (0.2 mmol) in acetonitrile (5 mL) at 80oC over 8 hours. After stirred for three hours, water (20 mL) was added and it was extracted with DCM (20 mL x 3). The combined organic layers were washed with brine (20 mL), dried over Na 2 SO 4 , filtered, and concentrated. Crude oil was obtained, which was used directly in the next step without further purification. To a solution of the above crude oil in THF (20 mL) at room temperature was added K 2 CO 3 (276 mg, 2.0 mmol, 2.0 equiv) and p -TsCl (0.22 mL, 1.5 mmol, 1.5 equiv) or 2,6-difluorophenylsulfonyl chloride (0.20 mL, 1.5 mmol, 1.5 equiv). After stirring for three hours, water (20 mL) was added and it was extracted with DCM (20 mL x 3). The combined organic layers were washed with brine (20 mL), dried over Na 2 SO 4 , filtered, and concentrated. 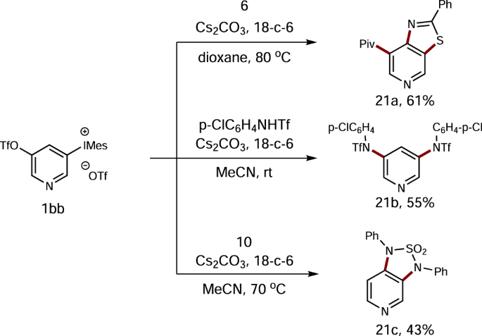Fig. 6: Study on pyridiyne precursor 1bb. All reactions are performed on a 0.2 mmol scale. Isolated yields are given. Flash column chromatography on silica gel afforded the corresponding 3-iodoaryl tosylate or 3-iodoaryl 2,6-difluorophenylsulfonate. General procedure for the oxidation of aryl iodides to form aryne precursors 1 (a) Oxidation with m -CPBA: To a solution of aryl iodide (1.0 mmol, 1.0 equiv) and TfOH (0.16 mL, 2.0 mmol, 2.0 equiv) in DCM (30 mL) at room temperature was added m -CPBA (190 mg, 1.1 mmol, 1.1 equiv). After stirred for 30 minutes, 1,3,5-trimethylbenzene (0.15 mL, 1.1 mmol, 1.1 equiv) was added. After three hours, all the volatiles were directly removed on a rotary evaporator. The resulting crude oil was triturated with diethyl ether and isolated by filtration to afford pure aryne precursor 1 . (b) Oxidation with Oxone: To a solution of aryl iodide (1.0 mmol, 1.0 equiv) and TfOH (0.16 mL, 2.0 mmol, 2.0 equiv) in MeCN (30 mL) at 0 °C was added Oxone (923 mg, 1.5 mmol, 1.5 equiv). After stirred for five minutes, 1,3,5-trimethylbenzene (0.15 mL, 1.1 mmol, 1.1 equiv) was added. After three hours, all the volatiles were directly removed on a rotary evaporator. The resulting crude oil was triturated with diethyl ether and isolated by filtration to afford pure aryne precursor 1 . General procedure for the synthesis of 1cc-1jj To a solution of compound 4 (0.22 mmol, 1.1 equiv) in anhydrous 2,2,2-trifluoroethyl alcohol (2 mL) at room temperature was added Koser’s reagent 5 (78.4 mg, 0.2 mmol, 1.0 equiv). After eight hours, it was filtrated. All the volatiles were then removed on a rotary evaporator. 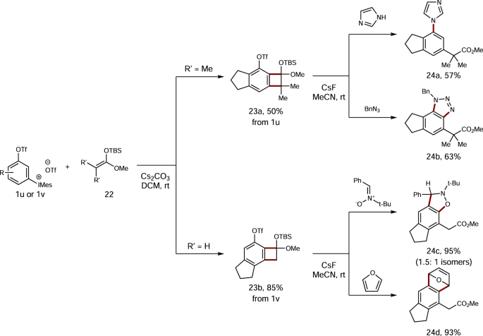Fig. 7: Manipulation through [2 + 2]-cycloaddition, Grob-fragmentation processes. All reactions are performed on a 0.4 mmol scale. Isolated yields are given. 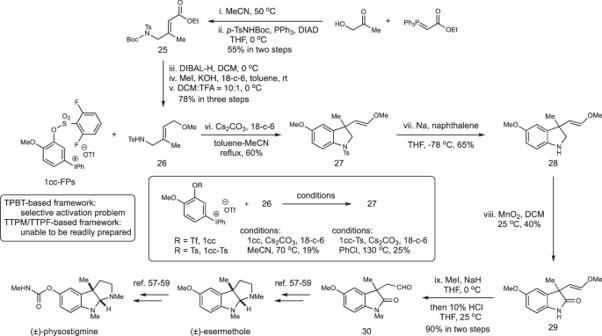Fig. 8: Study toward the synthesis of (±)-esermethole and (±)-physostigmine. A preparation of compound30was realized by employing domino aryne nucleophilic-ene reaction between aryne precursor1cc-FPsand compound26as the key step. After obtaining compound27, subsequent deprotection, oxidation, N-methylation, and conversion of the enol methyl ether to aldehyde gave rise to the desired compound30. Isolated yields are given. The resulting crude oil was triturated with diethyl ether and isolated by filtration to afford pure aryne precursor 1 .